Prediction of variable translation rate effects on cotranslational protein folding The concomitant folding of a protein with its synthesis on the ribosome is influenced by a number of different timescales including the translation rate. Here we present a kinetic formalism to describe cotranslational folding and predict the effects of variable translation rates on this process. Our approach, which utilizes equilibrium data from arrested ribosome nascent chain complexes, provides domain folding probabilities in quantitative agreement with molecular simulations of folding at different translation rates. We show that the effects of single codon mutations in messenger RNA that alter the translation rate can lead to a dramatic increase in the extent of folding under specific conditions. The kinetic formalism that we discuss can describe the cotranslational folding process occurring on a single ribosome molecule as well as for a collection of stochastically translating ribosomes. Ribosome-bound nascent protein chains are particularly vulnerable to misfolding and interacting in aberrant manners with other cellular components [1] . To avoid these potentially dangerous possibilities and facilitate the folding process [2] , a variety of quality control mechanisms are associated with translating ribosomes, including those involving molecular chaperones and other ancillary factors [1] . An additional level of control is provided by the opportunity for proteins to fold during synthesis [3] , [4] , [5] , [6] , thus potentially enhancing folding yields [7] and avoiding misfolded or intermediate species [8] , [9] . Given its importance, it is not surprising that the cotranslational folding process can be regulated by the modulation of the rates at which successive amino acids are covalently attached to the nascent chain during synthesis. Thus, for example, reduced folding yields have been observed when slow-translating messenger RNA codons are mutated to fast-translating codons [10] . Even single synonymous mutations have been reported to decrease the total enzymatic activity of specific types of proteins, presumably because of cotranslational misfolding [11] , leading to disease [12] . Furthermore, slow-translating codons have been observed to appear more frequently at domain boundaries [10] , which can result in increased folding yields. All these results indicate that the interplay of the timescales of domain folding and amino-acid addition to the nascent chain is crucial in determining the extent of cotranslational folding ( Fig. 1a ). 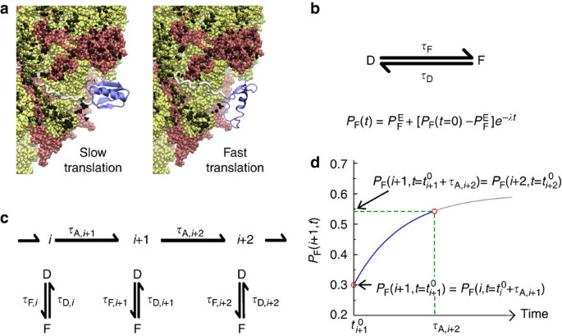Figure 1: Kinetic scheme for predicting variable translation rate effects on cotranslational folding. (a) Slower translation rates afford a protein domain (blue) more time to fold on the ribosome (left panel) than faster translation rates (right panel). Therefore, a slower translation rate is expected to increase the extent of cotranslational folding19,31. Ribosomal protein and RNA molecules are shown in red and yellow, respectively; the nascent chain's polyglycine linker is in white and the protein G domain is in blue. A portion of the ribosome has been removed in the figure to reveal the nascent chain in the exit vestibule. These structures were generated from continuous translation simulations with amino acids incorporated every 60 ms (left panel) and 1.3 ms (right panel). (b) A two-state model for protein interconversion between folded (F) and denatured (D) states, with mean folding and unfolding times denotedτFandτD.The time-dependence of folding,PF(t), is a function of these two timescales as well as the initial,PF(t=0), and final,PFE, folded fractions (λ=[τF]−1+[τD]−1). (c) A kinetic scheme for cotranslational folding. To make the two-state model applicable to cotranslational folding, we introduce the additional timescale,τA,i, of amino-acid addition of theith residue to the C-terminus of the nascent chain. The mean folding and unfolding times,τF,iandτD,i, depend explicitly on the nascent chain lengthi, and addition of a new amino acid to the nascent chain, which occurs afterτA,ims, represents an irreversible reaction. (d) Probability that the domain is folded at a timetand corresponding nascent chain lengthi+1 (PF(i+1,t)). For a two-state system, this probability relaxes towards its equilibrium value. The time available for folding at lengthi+1(that is, the dwell time) is equal to the timeτA,i+2it takes to incorporate thei+2 amino acid (see green dashed line). The final probability of folding at lengthi+1 is equal to the initial probability of folding at nascent chain lengthi+2, that is, Figure 1: Kinetic scheme for predicting variable translation rate effects on cotranslational folding. ( a ) Slower translation rates afford a protein domain (blue) more time to fold on the ribosome (left panel) than faster translation rates (right panel). Therefore, a slower translation rate is expected to increase the extent of cotranslational folding [19] , [31] . Ribosomal protein and RNA molecules are shown in red and yellow, respectively; the nascent chain's polyglycine linker is in white and the protein G domain is in blue. A portion of the ribosome has been removed in the figure to reveal the nascent chain in the exit vestibule. These structures were generated from continuous translation simulations with amino acids incorporated every 60 ms (left panel) and 1.3 ms (right panel). ( b ) A two-state model for protein interconversion between folded (F) and denatured (D) states, with mean folding and unfolding times denoted τ F and τ D. The time-dependence of folding, P F ( t ), is a function of these two timescales as well as the initial, P F ( t =0), and final, P F E , folded fractions ( λ =[ τ F ] −1 +[ τ D ] −1 ). ( c ) A kinetic scheme for cotranslational folding. To make the two-state model applicable to cotranslational folding, we introduce the additional timescale, τ A ,i , of amino-acid addition of the i th residue to the C-terminus of the nascent chain. The mean folding and unfolding times, τ F ,i and τ D ,i , depend explicitly on the nascent chain length i , and addition of a new amino acid to the nascent chain, which occurs after τ A, i ms, represents an irreversible reaction. ( d ) Probability that the domain is folded at a time t and corresponding nascent chain length i +1 ( P F ( i +1, t )). For a two-state system, this probability relaxes towards its equilibrium value. The time available for folding at length i+1 (that is, the dwell time) is equal to the time τ A ,i+ 2 it takes to incorporate the i +2 amino acid (see green dashed line). The final probability of folding at length i +1 is equal to the initial probability of folding at nascent chain length i +2, that is, Full size image Approaches based on the kinetic modelling of the molecular processes involved in translation have provided profound insights into the diverse functions of the ribosome. For example, the ability of the ribosome to discriminate between cognate and near-cognate transfer RNA has been explained using kinetic equations [13] , [14] . Here we extend this strategy to the prediction of the extent of nascent chain folding during continuous translation. This approach is based on the use of data on folding kinetics from arrested ribosome nascent chain (RNC) complexes and the time required to add individual residues to the nascent chain, quantities that can be measured using fluorescence or single molecule methods [15] , [16] . Making predictions based on arrested (that is, equilibrium) RNC data is convenient, because it is experimentally easier to probe such systems as compared with RNCs undergoing continuous, non-equilibrium translation [17] . Our approach is applicable to both single molecule and bulk cotranslational folding occurring during continuous protein synthesis. The extent of cotranslational folding on a single ribosome To develop our approach, we first note that, in many instances, the folding of protein domains consisting of less than about 100 residues often occurs in bulk solution without significantly populating any intermediate state, and hence can be described phenomenologically by a two-state model [18] ( Fig. 1b ). In this scheme, a protein can interconvert between folded (F) and denatured (D) states. In what follows, we will consider this model in the context of a translating protein, allowing us to predict the extent of cotranslational folding at different rates of translation. Translation introduces the additional timescale, τ A , of amino-acid addition to the two-state kinetic scheme ( Fig. 1c ). Because the chemical environment surrounding a protein domain changes, as it is synthesized, the timescales of its folding ( τ F ,i ) and unfolding ( τ D ,i ) are a function of the nascent chain length i , that is, the number of residues comprising the nascent chain at a particular point during its synthesis [4] . The time available for the domain to interconvert between folded and denatured states at length i is equal to τ A ,i +1 , corresponding to the time it takes to attach the amino-acid i +1 to the nascent chain. τ A ,i+ 1 has been shown to be influenced by a number of factors including the identity of the mRNA codon [19] , the intracellular concentration of cognate and near-cognate amino-acyl-tRNAs [20] , and the presence of secondary structure within the substrate mRNA [21] . For an apparent two-state folding protein, larger τ A,i+ 1 values will increase the probability P F ( i,t ) that the domain will fold (that is, achieve its native structure) by affording the domain more time to do so at a nascent chain length i and time t after initiation of synthesis ( Fig. 1d ). To derive an equation relating these three timescales ( τ A ,i+ 1 , τ F ,i , τ D ,i ) we first consider the behaviour of a single ribosome translocating along an mRNA molecule, and the time dependence of its nascent chain length. At a given nascent chain length i , the ribosome will dwell at codon i +1 waiting for this codon's cognate tRNA to be selected from the cytosol of the cell. This selection process involves a number of steps and a range of associated molecules such as elongation factor thermo unstable (EF-Tu). As we are concerned specifically with the nascent chain's length dependence as a function of time, we do not need to consider explicitly the details of these other chemical steps, for the reasons that follow. The time it takes to select the cognate tRNA and accommodate it into the A-site of the ribosome structure is stochastic in nature, but, on average, it is estimated in Escherichia coli to range from tens to hundreds of milliseconds depending on the identity of the tRNA molecule [20] . Once the A-site and P-site tRNAs are aligned, and receive sufficient thermal energy to pass over the transition state barrier, the chemical step of peptide bond formation, which changes the nascent chain length from i to i +1, takes on the order of picoseconds to nanoseconds [22] and is known as the transition path time [23] , [24] . This six orders-of-magnitude separation in the transition path time and τ A timescales (picoseconds versus milliseconds) means that, for an individual ribosome molecule, the transition from nascent chain length i to i +1 appears instantaneous relative to the time the ribosome spends at either of these chain lengths. As a consequence, the probability, P ( i ), that this single ribosome molecule will contain a nascent chain of length i at time t is equal to the boxcar function probability distribution which equals 1 in the time interval [ t i 0 , t i 0 + τ A,i+ 1 ) and is zero otherwise ( Fig. 2a ). t i 0 is the time at which the i th amino acid is added to the nascent chain after initiation of translation. 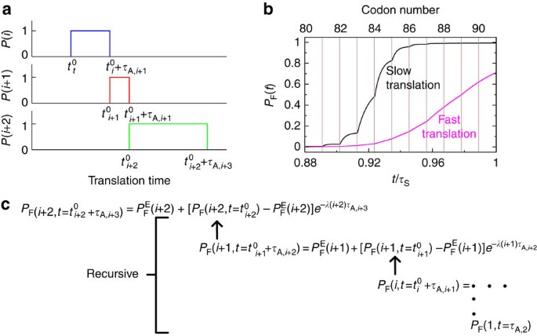Figure 2: Aspects of translation that are relevant in the derivation of the kinetic equation discussed in this work. (a) Probability of a single ribosome molecule containing a nascent chain length of (from top to bottom)i,i+1, andi+2 residues as a function of time. Because of the large separation of timescales between the chemical step of peptide bond formation and the ribosome dwell time at a specific codon, this probability is best approximated as a Boxcar function as shown. (b) Probability of the protein G domain folding as a function of the synthesis time and codon number (top axis) with new amino acids incorporated every 60 ms (black line) and 1.3 ms (magenta line). The equality of the initialPF(i+2,t=t01+2) and the finalPF(i+1,t=t0i+1+τA,i+2) folding probabilities can be clearly seen in this figure. These curves were predicted according to equation (4) based on protein G's folding and unfolding kinetics. To facilitate the comparison of folding at these two different synthesis rates, the time has been divided by their respective total synthesis time(c) Because of this equality, the folding behaviour ati+2 depends recursively on the behaviour at shorter nascent chain lengths. This is illustrated here by the kinetic equations that describe relaxation towards equilibrium (compare withFig. 1b), with each successive nascent chain length being a function (indicated by the arrows) of the relaxation behaviour at earlier times (that is, at shorter nascent chain lengths) during synthesis. This recursive relation is expressed compactly in equation (4). The change in P ( i ) with respect to time is Figure 2: Aspects of translation that are relevant in the derivation of the kinetic equation discussed in this work. ( a ) Probability of a single ribosome molecule containing a nascent chain length of (from top to bottom) i , i +1, and i +2 residues as a function of time. Because of the large separation of timescales between the chemical step of peptide bond formation and the ribosome dwell time at a specific codon, this probability is best approximated as a Boxcar function as shown. ( b ) Probability of the protein G domain folding as a function of the synthesis time and codon number (top axis) with new amino acids incorporated every 60 ms (black line) and 1.3 ms (magenta line). The equality of the initial P F ( i +2, t = t 0 1+2 ) and the final P F ( i +1, t = t 0 i +1 + τ A ,i+ 2 ) folding probabilities can be clearly seen in this figure. These curves were predicted according to equation (4) based on protein G's folding and unfolding kinetics. To facilitate the comparison of folding at these two different synthesis rates, the time has been divided by their respective total synthesis time ( c ) Because of this equality, the folding behaviour at i +2 depends recursively on the behaviour at shorter nascent chain lengths. This is illustrated here by the kinetic equations that describe relaxation towards equilibrium (compare with Fig. 1b ), with each successive nascent chain length being a function (indicated by the arrows) of the relaxation behaviour at earlier times (that is, at shorter nascent chain lengths) during synthesis. This recursive relation is expressed compactly in equation (4). Full size image where δ ( t ) is the Dirac delta function centred at time t after initiation of translation ( Fig. 2a ). Next, we note that the experimentally observed timescale of the folding and unfolding process of a protein domain in free solution is typically on the order of milliseconds or more [25] , and may be much longer near the ribosome surface [26] . Therefore, the picosecond-to-nanosecond transition-path time of peptide bond formation will also appear as instantaneous relative to the milliseconds or more folding/unfolding timescale. As a consequence, the probability that the nascent chain is in the folded state is equal immediately before (denoted P F ( i,t = t i 0 + τ A ,i+ 1 )) and immediately after (denoted P F ( i +1, t = t i +1 0 )) the addition of the i +1 amino acid ( Fig. 1d ); that is, the starting point of folding at length i +1 is equal to the ending point at length i . Thus, during continuous translation, the extent of folding at a given nascent chain length is a function of the extent of folding at shorter lengths, and, hence, cotranslational folding depends recursively on what has happened at earlier times during the synthesis of the protein ( Figs. 2b,c ). As translation is a non-equilibrium process, memory effects can become prevalent, and so it is not surprising that the extent of cotranslational domain folding depends on the states populated at earlier times during synthesis ( Fig. 2c ). The specific behaviour of a single ribosome translocating along an mRNA containing N codons is therefore characterized by the series of dwell times at each codon If we have many independent measurements of domain folding on ribosomes that exhibit the same series of dwell times, then we can treat the domain folding probability as continuous and write down the differential equation defining the domain folding probability with respect to time as and its solution is We substitute equation (3) into the recursive equations shown in Fig. 2c and rearrange them to find that P F at arbitrary nascent chain length i and time t is In equations (3) and (4), is the equilibrium probability of folding and equals with λ ( i ) being the rate of interconversion of the folded and denatured states that equals [ τ F,i ] −1 +[ τ D ,i ] −1 . This is in contrast to the out-of-equilibrium quantity in equation (3), which is the folding probability immediately after adding the i th residue to the nascent chain. τ F ,i and τ D ,i are the average times of folding and unfolding at nascent chain length i on an arrested RNC. The placement of the first residue ( i =1) in the P-site of the ribosome, corresponding to fmet -tRNA in prokaryotes [27] , is designated as time point zero, t 1 0 =0 s, and the time at which the i th residue is added is Accurate prediction of individual codon translation rate effects Equation (4) is a function solely of τ F,i , τ D ,i , τ A ,i and is a closed form solution to differential equations (1) and (2); therefore it provides an exact solution to the kinetic model shown in Fig. 1c . This equation expresses the probability that a domain is folded at each codon during continuous translation in terms of the equilibrium quantities and λ ( i ) that can be measured on arrested ribosomes, and the translation time of each codon ( τ A,i ), which can be measured by FRET and laser optical tweezer methods [15] , [16] . To date, however, few such measurements at different nascent chain lengths have been reported. Therefore, to test equation (4) rigorously, we generated an independent data set representing the probability of domain folding at various translation rates using coarse-grained molecular simulations ( Supplementary Methods ) of the synthesis of protein G on the ribosome from Thermus thermophilus ( Fig. 1a ). Protein G is a single domain protein whose folded architecture consists of an α-helix located adjacent to a four-stranded β-sheet platform [28] . The coarse-grained model that we use has been shown previously to be consistent with a range of experimental data from arrested RNC complexes [4] , [29] . As in analogous experiments [17] , we attached an unstructured linker to the carboxy terminus of protein G ( Fig. 3a ) to allow folding and unfolding of this domain to occur near the exit tunnel vestibule, where nascent chain tertiary interactions are sterically permitted [29] , [30] . 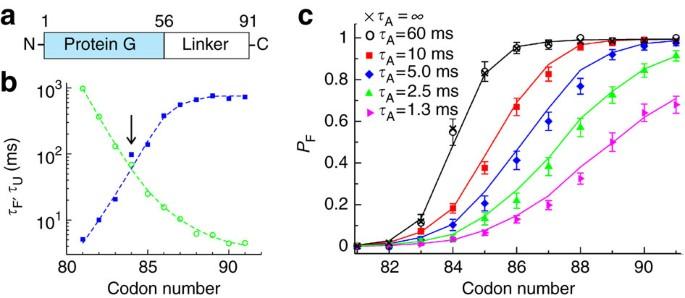Figure 3: Probability of cotranslational folding as a function of the translation rate. (a) To test the accuracy of the kinetic model (equation (4)), we simulated protein G as a RNC using a well-established coarse-grained model4,29(Supplementary Methods). We attached a polyglycine linker (codons 57 to 91) to the C-terminus of protein G (codons 1 to 56) to allow it to fold and unfold near the exit tunnel vestibule. (b) Average folding (τF, green circles) and unfolding (τU, blue squares) times as a function of nascent chain length on an arrested ribosome (τA=∞) calculated from the coarse-grained Langevin dynamics simulations (s.e.m. is shown for 15 replicates). The arrow indicates the nascent chain length at which the domain is folded with close to 50% probability. Lines are to guide the eye and are not based on any model. (c) Probability of domain folding during continuous translation as a function of nascent chain length (s.e.m. is shown for 5 replicates). Amino-acid incorporation timescales range from 1 to 60 ms and are constant for a given system. Equilibrium data are shown by blackxsymbols. The results from the coarse-grained simulations are shown as symbols, while the predictions from equation (4) are shown as solid lines and utilize the data from (b) as its arguments. ThePFdata shown were calculated immediately before addition of the next amino acid to the nascent chain. Figure 3: Probability of cotranslational folding as a function of the translation rate. ( a ) To test the accuracy of the kinetic model (equation (4)), we simulated protein G as a RNC using a well-established coarse-grained model [4] , [29] ( Supplementary Methods ). We attached a polyglycine linker (codons 57 to 91) to the C-terminus of protein G (codons 1 to 56) to allow it to fold and unfold near the exit tunnel vestibule. ( b ) Average folding ( τ F , green circles) and unfolding ( τ U , blue squares) times as a function of nascent chain length on an arrested ribosome ( τ A =∞) calculated from the coarse-grained Langevin dynamics simulations (s.e.m. is shown for 15 replicates). The arrow indicates the nascent chain length at which the domain is folded with close to 50% probability. Lines are to guide the eye and are not based on any model. ( c ) Probability of domain folding during continuous translation as a function of nascent chain length (s.e.m. is shown for 5 replicates). Amino-acid incorporation timescales range from 1 to 60 ms and are constant for a given system. Equilibrium data are shown by black x symbols. The results from the coarse-grained simulations are shown as symbols, while the predictions from equation (4) are shown as solid lines and utilize the data from ( b ) as its arguments. The P F data shown were calculated immediately before addition of the next amino acid to the nascent chain. Full size image We first calculated the equilibrium folding and unfolding kinetics (that is, τ F ,i and τ D ,i ) of protein G on arrested RNCs containing nascent chain lengths ranging from 81 to 92 AA ( Fig. 3b ). These timescales can be seen to vary with the nascent chain length, a result attributable to the change in chemical environment around the domain that arises in the simulations from electrostatic and excluded volume interactions between the nascent chain and the ribosome surface. We then simulated the continuous translation of protein G by covalently attaching new glycine residues to the nascent chain's C terminus at the biologically relevant [20] constant time intervals of 60, 10, 5, 2.5, and 1.3 ms, starting from a nascent chain length of 71 AA; at this length, protein G is unfolded on the ribosome as the C-terminal portion of the domain is in the exit tunnel [4] . To obtain statistically significant results, we carried out between 32 and 384 independent protein synthesis simulations at each translation rate. The effects of translation rate on the extent of protein G folding at each nascent chain length are shown in Fig. 3c , and the corresponding root-mean-squared deviations of the protein G domain from its X-ray structure are shown in Fig. 4 . We observe, consistent with previous conjectures [31] , that the greater the translation rate the smaller the probability that the domain is folded at a given nascent chain length. Furthermore, at synthesis times close to the average value in E. coli , that is, τ A =50 ms, we find that continuous translation and arrested RNCs result in the same extent of folding as a function of nascent chain length ( Fig. 3c ). This result occurs because the folding of protein G, during continuous translation at τ A =60 ms, occurs under quasi-equilibrium conditions, where the folding reaction is under thermodynamic control, whereas at τ A =1.3 ms cotranslational folding occurs under non-equilibrium conditions, where folding is under kinetic control [4] . It is important to emphasize that domains that fold on timescales of greater than 50 ms are more likely to be under kinetic control at synthesis timescales of τ A ≤50 ms ( τ F =2 ms for protein G in free solution [25] ), and hence show a deviation between the non-equilibrium and equilibrium folding curves P F ( i, t ) and . In a database of single domain folding timescales [25] under physiologically relevant conditions, a quarter of them have τ F ≥50 ms. Thus, at average E. coli synthesis rates during exponential growth [32] , cotranslational folding of 25% or more of domains in multidomain proteins may be under kinetic control. 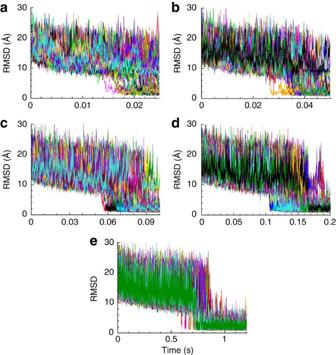Figure 4: Root-mean-squared deviation of the protein G domain. Root-mean-squared deviation of the protein G domain from its X-ray structure (PDB code 1GB1) during its continuous translation on the ribosome as a function of the simulation time (mapped onto the experimental timescale—seeMethods). Each independent synthesis trajectory is shown as a different colour. Time equal to zero corresponds to a nascent chain length of 72 residues; the final nascent chain length is 91 residues. Panels (a) through (e) correspond, respectively, to adding a glycine to the C-terminal nascent chain residue every 1.3, 2.5, 5, 10, 60 ms. Figure 4: Root-mean-squared deviation of the protein G domain. Root-mean-squared deviation of the protein G domain from its X-ray structure (PDB code 1GB1) during its continuous translation on the ribosome as a function of the simulation time (mapped onto the experimental timescale—see Methods ). Each independent synthesis trajectory is shown as a different colour. Time equal to zero corresponds to a nascent chain length of 72 residues; the final nascent chain length is 91 residues. Panels ( a ) through ( e ) correspond, respectively, to adding a glycine to the C-terminal nascent chain residue every 1.3, 2.5, 5, 10, 60 ms. Full size image Importantly for the purpose of this study, the data in Fig. 3c provide a means to test the accuracy of equation (4). Inserting the arrested RNC folding kinetics from Fig. 3b into equation (4) and setting τ A to the corresponding value used in the simulations, we find this kinetic formalism accurately and rapidly predicts the extent of cotranslational folding as a function of the translation rate ( Fig. 3c ). Thus, our approach captures the interplay of translation rate and folding and denaturation timescales and its consequence for the extent of cotranslational folding. To test the sensitivity of equation (4) to single codon mutations that locally alter the translation rate along an mRNA molecule, we simulated cotranslational folding of protein G when a single 'fast'-translating codon ( τ A,87 =1.3 ms) was placed at codon 87 in the context of a 'slow'-translating mRNA sequence ( τ A =10 ms). Conversely, we also simulated a system in which a single 'slow'-translating codon ( τ A,90 =10 ms) was placed at codon 90 in the context of a 'fast'-translating mRNA sequence ( τ A =1.3 ms). We find that equation (4) accurately predicts the change in the extent of domain folding that results from the change in single synonymous codon mutations ( Fig. 5a ). This is a crucial demonstration of the utility of this formalism as synonymous mutations have been shown to alter folding yields dramatically [19] . These results also demonstrate that the predictions from this kinetic formalism are accurate and sensitive to the effect of variable translation rates at the level of single codons. 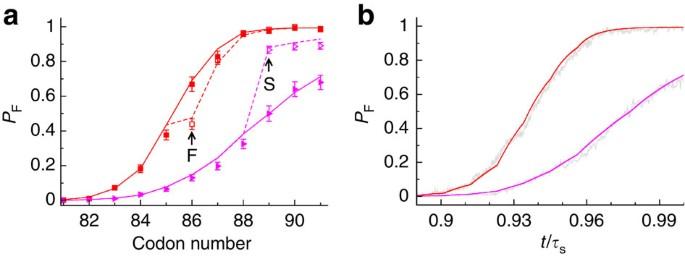Figure 5: The effects of synonymous codon mutations on cotranslational folding are accurately predicted by equation (4). (a) Comparison of the probability of protein G domain folding during continuous translation with amino acids added everyτA=10 ms (solid red squares) andτA=1.3 ms (solid magenta triangles). The s.e.m. is shown for five replicates. A single fast translating codon, withτA,87=1.3 ms, was inserted at codon 87 (which shortens the dwell time at position 86 indicated by an arrow and the letter 'F') of the slower translating system (τA=10) and its effect onPFis shown by the open red squares and the dashed red line. A single slower translating codon, withτA,90=10 ms, was inserted at codon 90 (indicated by an arrow and 'S') of the faster translating system (τA=1.3 ms) and its effect onPFis shown by the open magenta triangles and the dashed magenta line. Coarse-grained simulation results are shown as symbols and predictions from equation (4) are shown as solid and dashed lines. In all systems, the final amino-acid sequence was the same. (b) Folding probability of the protein G domain as a function of the translation time for the slow (red line,τA=10) and fast (magenta line,τA=1.3 ms) translating mRNA. For each system, the time has been scaled by their total synthesis time. The predictions from equation (4) are shown as coloured lines and the results from the continuous translation simulations of the coarse-grained model are shown in grey. The difference in the absolute scaleτSmeans that there are less data points for the fast translating mRNA system, making the simulation data appear less noisy. Figure 5: The effects of synonymous codon mutations on cotranslational folding are accurately predicted by equation (4). ( a ) Comparison of the probability of protein G domain folding during continuous translation with amino acids added every τ A =10 ms (solid red squares) and τ A =1.3 ms (solid magenta triangles). The s.e.m. is shown for five replicates. A single fast translating codon, with τ A,87 =1.3 ms, was inserted at codon 87 (which shortens the dwell time at position 86 indicated by an arrow and the letter 'F') of the slower translating system ( τ A =10) and its effect on P F is shown by the open red squares and the dashed red line. A single slower translating codon, with τ A,90 =10 ms, was inserted at codon 90 (indicated by an arrow and 'S') of the faster translating system ( τ A =1.3 ms) and its effect on P F is shown by the open magenta triangles and the dashed magenta line. Coarse-grained simulation results are shown as symbols and predictions from equation (4) are shown as solid and dashed lines. In all systems, the final amino-acid sequence was the same. ( b ) Folding probability of the protein G domain as a function of the translation time for the slow (red line, τ A =10) and fast (magenta line, τ A =1.3 ms) translating mRNA. For each system, the time has been scaled by their total synthesis time. The predictions from equation (4) are shown as coloured lines and the results from the continuous translation simulations of the coarse-grained model are shown in grey. The difference in the absolute scale τ S means that there are less data points for the fast translating mRNA system, making the simulation data appear less noisy. Full size image While the folding probabilities are shown as a function of nascent chain length in Figs 3c and 5a , equation (4) can also accurately predict these folding curves as a function of the time after the initiation of translation ( Fig. 5b ). Application to a collection of translating ribosomes In the preceding treatment, we considered a single ribosome molecule translocating along an mRNA molecule. Equation (4) therefore represents the average domain folding probability of a nascent chain on a ribosome that translocates with a specific series of dwell times { τ A }. As translocation of a ribosome along mRNA is stochastic, with a distribution of amino-acid addition times at a codon i , experiments on different ribosomes can yield different series of dwell times while they translate the same mRNA sequence. How can we combine the exact result of equation (4), which utilizes a specific series of dwell times, with the stochastic nature of an ensemble of ribosomes, each with their own respective series of dwell times? If the probability density function P i ( τ A ) of amino-acid addition times at codon i is known a priori , then for a specific series of N dwell times, labelled as set k ({ τ A } k ), we can calculate the probability p k of that series occurring by random chance as Therefore, by inserting the same series of dwell times in both equations (4) and (5) , and multiplying the result as p k P F ( i = N , t N 0 + τ A ,i+ 1 ), we obtain the contribution of the P F ( i ) folding curve of a single translating ribosome (for example, Fig. 3c ) to the folding curve that would result from averaging over a large number of independent, stochastically translating ribosomes. This result is useful for three reasons. First, equation (5) allows for the calculation of the probability of obtaining a particular single molecule trace (defined by the set of dwell times) in an experiment. Second, it allows for the numerical simulation of an arbitrarily large number of independent, stochastically translating ribosomes and each of their corresponding cotranslational folding probability curves. And finally, with sufficient such simulations, the distribution of folding probability curves and their average can be calculated for an ensemble of stochastically translating ribosomes. Importantly, this approach can be applied to arbitrary P i ( τ A ) distributions, thus providing it significant versatility. To illustrate these points, consider an amino-acid addition time distribution P i ( τ A ) that is exponentially distributed and is therefore equal to where ‹ τ A,i+ 1 › is the average time required for amino-acid addition to a nascent chain of length i . Values of this time have already been estimated for all 48 codons in E. coli [20] . τ k A ,i +1 is the time it takes to add the i +1 residue to the nascent chain in the k th experiment in which a single ribosome translocating along mRNA is monitored. If N =91, as in the protein G construct discussed above, and ‹ τ A ,i+ 1 › is taken as 60 ms for all codons, then the probability of observing a single ribosome translate a protein in which it dwells at each codon for 20 ms is effectively zero (about 10 −171 ). To simulate the individual folding curves of 1,000 ribosomes stochastically translating this protein G construct; however, we can randomly sample τ A values from the exponentially distributed P i +1 ( τ A ) for each codon (see Methods ) and construct 1,000 unique dwell time sets [{ τ A } k ]. For each τ A set, we can use equation (4) to calculate the resulting folding curve. Fig. 4 shows these 1,000 folding curves as a function of time ( Fig. 6a ) and nascent chain length ( Fig. 6b ). These results show that the kinetic model that we described can be utilized to predict how amino-acid timescales and their underlying distribution affect the extent of cotranslational folding of a protein domain at the resolution of an individual ribosome molecule, or for a large collection of ribosomes. 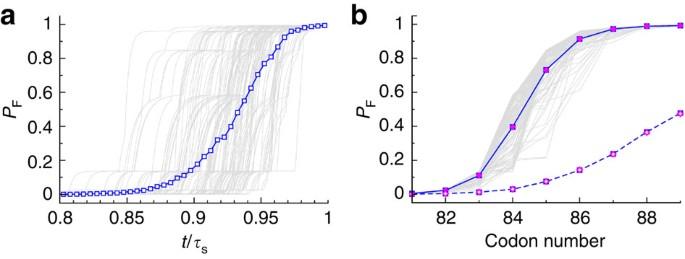Figure 6: Behaviour of a collection of stochastically translating ribosomes. (a) Cotranslational folding probability of protein G as a function of time for 110 stochastically translating ribosomes (grey lines). The variation in behaviour arises from the different series of dwell times {τA} associated with each ribosome. The blue line is the folding probability averaged over 1,000 such stochastically translating ribosome molecules. These data were numerically simulated by assumingPi(τA) is exponentially distributed with ‹τA,i›=60 ms for alli(seeMethods). (b) Same as (a), except that the folding probability is shown per codon number immediately before the addition of the next residue to the nascent chain. Additionally, the ensemble average assuming ‹τA,i›=1.3 ms for alliis also shown as a dashed blue line and squares. Predictions from equation (6) are shown as filled and open magenta diamonds for ‹τA,i›=60 ms and 1.3 ms, respectively. Figure 6: Behaviour of a collection of stochastically translating ribosomes. ( a ) Cotranslational folding probability of protein G as a function of time for 110 stochastically translating ribosomes (grey lines). The variation in behaviour arises from the different series of dwell times { τ A } associated with each ribosome. The blue line is the folding probability averaged over 1,000 such stochastically translating ribosome molecules. These data were numerically simulated by assuming P i ( τ A ) is exponentially distributed with ‹ τ A ,i › =60 ms for all i (see Methods ). ( b ) Same as ( a ), except that the folding probability is shown per codon number immediately before the addition of the next residue to the nascent chain. Additionally, the ensemble average assuming ‹ τ A ,i › =1.3 ms for all i is also shown as a dashed blue line and squares. Predictions from equation (6) are shown as filled and open magenta diamonds for ‹ τ A ,i ›=60 ms and 1.3 ms, respectively. Full size image Exact solution for a collection of ribosomes When P i +1 ( τ A ) is exponentially distributed, it is possible to derive an exact expression relating the average cotranslational folding curve from a collection of stochastically translating ribosomes as a function of nascent chain length (equation (6), Attila Szabo, personal communication). That is, the blue line in Fig. 6b can be predicted without having to resort to the numerical simulations discussed in the previous section, although, by doing so, the information on the underlying distribution of folding curves is lost. To derive the ensemble averaged folding curve as a function of nascent chain length, denoted ‹ P F ( i )›, a probabilistic approach can be utilized to analyse the elementary reaction steps in Fig. 1c (see Methods ). Under these conditions, where the superscript of '−1' indicates the reciprocal of these timescales. To test the accuracy of equation (6), we used it to calculate ‹ P F ( i )› for protein G and compared it with results from the numerical simulations described in the previous section. We find excellent agreement between this exact result and the numerical simulations ( Fig. 6b ). Thus, equation (6) can predict the effect of per codon translation rates on the average cotranslational folding curve that arises from bulk experiments. We have presented two equations (equations (4) and (6)) that predict the extent of cotranslational domain folding based on per codon translation timescales, and the timescales of domain folding and denaturation on arrested RNC complexes at equilibrium ( Fig. 3b ). We have derived an exact expression for the domain folding probability in the case of a single translating ribosome (equation (4)), and shown how this expression can be utilized to predict the behaviour of a large number of stochastically translating ribosomes. Finally, an exact expression for the cotranslational folding curve was derived for ribosomes translating with exponential dwell times at each codon (equation (6)). The utility of each of these equations depends on the questions that one is interested in addressing and the type of experiment (bulk versus single molecule) that is being carried out. In analysing and predicting cotranslational folding behaviour on individual ribosomes, equation (4) is perhaps the most relevant. The application, via numerical methods, of equation (4) to a collection of stochastically translating ribosomes is of direct consequence to both single molecule and bulk experiments as this approach offers the ability to calculate the individual ribosome folding curves as well as the ensemble average. This numerical approach can handle arbitrary distributions of amino-acid addition timescales and is thus not limited to the exponential dwell time distributions. Bulk experiments, where the average cotranslational folding curve as a function of nascent chain length may be measured from a collection of ribosomes, can be predicted using equation (6). Thus, these equations are applicable under a wide range of conditions. Laser optical tweezers have recently [26] been used to measure the folding rate under tension of T4-lysozyme arrested on the ribosome at two different linker lengths. While the unfolding rate at zero force was not estimated at either length, these experiments clearly demonstrate that it is possible to measure τ F ,i and τ D ,i experimentally, which are key inputs in our approach. We expect that, as more studies measuring these rates are carried out on this and other proteins, such data, when combined with our approach, will be useful in predicting what happens during continuous translation. A number of additional translation-associated processes were not explicitly considered in the reaction scheme ( Fig. 1c ). For example, the competitive (and reversible) binding of near- and non-cognate tRNAs for a codon can slow down the rate of amino-acid addition by cognate tRNA molecules [20] . Furthermore, chaperones such as trigger factor directly interact with nascent chains during their synthesis, and can slow the rate of cotranslational folding of at least some proteins [33] . These processes do not diminish the utility of our approach, because each of these additional processes can effectively be accounted for by incorporating them into the timescales of amino-acid addition (in the case of competitive binding) and into the rates of folding and unfolding (in the case of trigger factor). The mathematical dependence of τ A on near-cognate and non-cognate tRNA concentrations and their competitive binding rates has been worked out previously [20] . Thus, combining that model with equation (4) provides a means to model the effect of competitive tRNA binding on cotranslational folding. Similarly, when quantitative experimental measurements become available for the effect of trigger factor on the rates of domain folding and unfolding, they can be incorporated implicitly into effective timescales in these equations. The kinetic models that we have described here are based on domains that fold cotranslationally in a two-state manner. This property applies to a variety of small proteins (typically ≤100 residues) and enables an analytical solution to be obtained for the kinetics of cotranslational folding. For protein domains larger than those examined here, which may populate intermediate states on the ribosome, the kinetic scheme in Fig. 1c can be modified to account for such additional states as they are experimentally identified. Although the additional complexity of such kinetic schemes may make it difficult to find an analytical solution, they could always be solved by numerical methods. The approach we have proposed here has many potential applications in the areas of in vivo protein folding, biotechnology, and synthetic biology. For example, when coupled with models of translation rates that account for codon usage and tRNA concentrations [34] , this formalism provides a means to predict cotranslational folding behaviour of entire proteomes under varying cellular conditions and aid in the design and of synthetic transcriptomes that optimize the extent of cotranslational folding. Equations (4) and (6) also provide a way for experimentalists to map directly the results from more easily studied arrested RNCs to the realistic situation of continuous translation. Thus, such kinetic modelling of the ribosome, when combined with a variety of different experimental data, provides new research avenues and the potential for novel insights in a number of different areas. An exact solution for a collection of translating ribosomes An equation can be derived relating the domain folding probability immediately before the addition of the next amino acid to the nascent chain for a ribosome that dwells with an exponential waiting time distribution at each codon (equation (6), Attila Szabo, personal communication). This probability, denoted is equal to the probability of taking the pathway in Fig. 1c F i →F i +1 and can be calculated as where and are, respectively, the probabilities that, when the nascent chain changes from length i −1 to i , the domain was either in the folded or denatured state. is the probability, that, beginning in the folded state at length i , the RNC complex will reach the folded state at length i +1 before reaching the denatured state at length i +1. Likewise, is the probability that, beginning in the denatured state at length i , the system will reach the folded state at length i +1 before reaching the denatured state at length i +1. Because there are only two states in our reaction scheme ( Fig. 1c ), we have that Substituting this into equation (7), we have and we see that is a recursive relationship. Using the probabilistic method [35] for calculating pathway probabilities in reaction schemes, and can be easily shown to equal, respectively, and Inserting these terms into equation (8), and using the boundary condition that at i =1 (that is, for a nascent chain comprising one residue, the domain is denatured), this recursive relationship when solved equals equation (6). Numerical simulation of a collection of translating ribosomes To simulate the stochastic nature of translation, it is necessary to consider the randomly distributed dwell times { τ A } that the ribosome exhibits during its translation of an mRNA molecule. As the underlying P i ( τ A ) distribution of amino-acid addition times at codon i has not yet been experimentally determined, here we assume it to be exponentially distributed with For each ribosome, we constructed its { τ A } by randomly sampling from this distribution, using an inverse transform sampling in which where R is a random number selected from a uniform distribution in the range of (0,1). For each ribosome, this procedure results in 91 dwell times, representing a ribosome stochastically translating the protein G construct ( Fig. 3a ). This procedure was repeated 1,000 times, each yielding a unique { τ A }, which represents the behaviour of 1,000 different synthesis events of this protein. Each { τ A } was then inserted into equation (4) to yield their corresponding cotranslational folding curve ( Fig. 6 ). Analysis of coarse-grained simulations Mapping simulation timescales to experimental timescales. Low viscosity Langevin dynamics, as used in the coarse-grained simulations ( Supplementary Methods ), accelerate molecular dynamics while leaving the thermodynamic properties of the system unaltered. To map these accelerated kinetics to the experimentally relevant high-viscosity situation in aqueous media, we multiply the simulation time by the constant the ratio of experimentally measured to calculated folding times. is the experimentally (E) measured folding time of protein G in bulk solution and equals 2.4 ms (ref. 25 ), whereas is the average folding time from these simulations in the absence of the ribosome and equals 3.6 ns. This constant represents a linear scaling between the simulation time and the experimental time. Thus, in these simulations, when a new glycine residue is inserted into the growing chain during continuous translation every 90 ns (=6×10 6 integration time steps) of simulation time, this interval corresponds to an experimental time of τ A =60 ms. Likewise, τ F , τ D and the other τ A values reported in the main text are the results of multiplying their simulation times by this constant. The probability of domain folding at equilibrium, P F E , was calculated from the Replica exchange simulations ( Supplementary Methods ). A given simulation conformation of protein G was considered to be folded, if its fraction of native contacts was greater than 50%, and otherwise was considered unfolded. The folded/unfolded time series for each replica was constructed using this definition, and the time series from replicas at different temperatures combined in the WHAM equations [36] to calculate P F E . The stability of the folded state of protein G with respect to its denatured state, ΔG ND , is equal to where k B is Boltzmann's constant and T is the temperature. The mean folding time τ F of protein G equals the average of the set of first passage times { τ F , i } determined from temperature quench simulations at various nascent chain lengths ( Supplementary Methods ). τ D is calculated as where k B is Boltzmann's constant and T is the simulation temperature. The probability of domain folding during continuous synthesis simulations, P F ( i ), was calculated as where the summation is over the N -independent trajectories simulated for the given system, θ ( Q BB , i −0.50) is the Heaviside step function that equals 1 if more than half of the native backbone contacts Q BB , i in the structure of protein G are made in the last frame of the simulation at nascent chain length i and 0 otherwise. where C is the number of native backbone contacts within the crystal structure, S (=56) is the number of interaction sites in protein G, and r jk F and r jk are, respectively, the spatial distances between interaction sites j and k in the crystal structure and the simulation structure. In this analysis, a native contact is identified in the crystal structure if any heavy atoms between residues j and k are within 4.5 Å of each other. The standard error about the mean of τ F was calculated by breaking the 152 independent folding trajectories into 15 sets of 10 or 11 τ F ,i values each, calculating the average value of each set and then calculating the standard deviation of the 15 averages divided by To calculate the s.e.m. of ΔG ND , the replica exchange simulation time-series data were broken into 5 independent sets, with approximately 20,000 points in each replica in each set. We then calculated ΔG ND using each data set in the WHAM equations, and calculated the s.e.m., using these five ΔG ND values. τ D 's s.e.m. was calculated using standard propagation of error equations. How to cite this article: O'Brien, E. P. et al . Prediction of variable translation rate effects on cotranslational protein folding. Nat. Commun. 3:868 doi: 10.1038/ncomms1850 (2012).